An insect-induced novel plant phenotype for sustaining social life in a closed system Foraging, defense and waste disposal are essential for sustaining social insect colonies. Hence, their nest generally has an open structure, wherein specialized castes called workers and soldiers perform these tasks. However, some social aphids form completely closed galls, wherein hundreds to thousands of insects grow and reproduce for several months in isolation. Why these social aphids are not drowned by accumulated honeydew has been an enigma. Here we report a sophisticated biological solution to the waste problem in the closed system: the gall inner surface is specialized for absorbing water, whereby honeydew is promptly removed via the plant vascular system. The water-absorbing closed galls have evolved at least twice independently among social aphids. The plant-mediated waste removal, which entails insect’s manipulation of plant morphogenesis and physiology, comprises a previously unknown mechanism of nest cleaning, which can be regarded as ‘extended phenotype’ and ‘indirect social behavior’ of the social aphids. Many insects form conspicuous galls on their host plants. The galls provide the inducer insects with isolated and exclusive habitat, constant and high-quality food supply, physical barrier against predators and parasites, and mitigated environmental stresses such as desiccation and temperature fluctuation [1] . The gall-forming insects manipulate the plant growth and morphogenesis for their own sake in a sophisticated manner, thereby inducing elaborate plant structures as ‘extended phenotypes’ of the insects [2] . Social insects such as bees, wasps, ants and termites generally form elaborate nests, in which some colony members reproduce, whereas other members do not necessarily participate in reproduction but comprise specialized castes called workers and soldiers. Foraging, defense and waste disposal are essential for sustaining social insect colonies. As the colony members constantly require a large amount of food from the environment and also produce a large amount of wastes to be disposed outside, the social insect colonies are generally unable to persist in isolation, and these altruistic individuals actively perform social tasks such as foraging, nursing, housekeeping, waste disposal, colony defense and so on [3] . Some aphids also produce altruistic individuals called soldiers, whose primary social role is usually defense, whereas some of them may also perform other social tasks such as waste disposal and gall repair [4] , [5] . Many, if not all, of them form conspicuous galls on their host plants and live socially therein. Aphids feed exclusively on plant phloem sap, and as gall tissue constantly supplies the inhabitants with plant sap, no foraging outside is needed for the gall-forming social aphids. On the other hand, waste disposal is an essential issue for them, because the gall inhabitants constantly produce large quantities of honeydew and other wastes. In many gall-forming social aphids, their galls have small openings, through which soldier nymphs actively dispose honeydew droplets and other colony wastes [6] , [7] , [8] , [9] , [10] , [11] , [12] . The enigma here is the presence of social aphids that form completely closed galls. Their galls remain closed for several months until their final dehiscence, and contain hundreds to thousands of insects. Their soldier nymphs may attack gall-boring predators that occasionally invade their galls, but do not perform gall cleaning [13] , [14] , [15] , [16] , [17] , [18] , [19] . It is expected that the large quantity of honeydew excreted by hundreds of aphids would quickly fill up the closed gall cavity. Aphid honeydew usually contains substantial quantities of sugars [20] , which may cause contamination and other problems in the aphid galls. Why doesn’t the watery waste drown and kill these social aphids confined in the closed galls? Here we report a sophisticated biological solution to the waste problem in the closed system: these social aphids have evolved to induce galls with an inner surface specialized for absorbing water, whereby honeydew waste is promptly removed via the plant vascular system. Our finding unveils a previously unknown mechanism of gall cleaning, which can be regarded as an ‘extended phenotype’ and a ‘plant-mediated social behavior’ of the social aphids with an imprisoned lifestyle. Phylogeny and gall formation of Hormaphidinae aphids The aphid subfamily Hormaphidinae consists of the tribes Nipponaphidini, Hormaphidini and Cerataphidini. On their primary host plants, these aphids form conspicuous galls that harbor hundreds, thousands or more colony members: closed galls on Distylium spp. by Nipponaphidini species; open galls on Hamamelis spp. by Hormaphidini species; and open galls on Styrax spp. by Cerataphidini species ( Fig. 1 ; Supplementary Fig. S1 ) [4] . Note that a Cerataphidini species, Ceratovacuna nekoashi, exceptionally forms a banana-shaped closed gall [15] . Most of the Hormaphidinae species produce soldier nymphs in their galls, which defend their galls against predators. In the species that form open galls, the soldier nymphs perform an additional social task for cleaning their galls: pushing wastes such as honeydew droplets, shed skins and dead insects out of the gall through the opening(s) [4] , [5] . In the species that form closed galls, by contrast, such a waste disposal is impossible for several months until the galls open upon maturity. 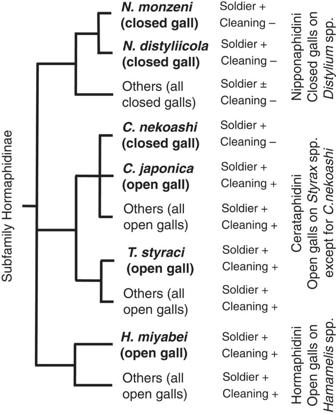Figure 1: A schematic phylogenetic relationship of the gall-forming social aphids. Species examined in this study representing the tribes Nipponaphidini, Hormaphidini and Cerataphidini of the subfamily Hormaphidinae are shown. Their gall type, soldier production and gall-cleaning behavior are mapped on the phylogeny. +, − and ± indicate presence of the trait, absence of the trait and some species with the trait while other species without the trait, respectively. Galls of six species examined in this study,N. monzeniandN. distyliicolafrom Nipponaphidini,C. nekoashi,C. japonicaandT. styracifrom Cerataphidini, andH. miyabeifrom Hormaphidini are indicated in bold. Figure 1: A schematic phylogenetic relationship of the gall-forming social aphids. Species examined in this study representing the tribes Nipponaphidini, Hormaphidini and Cerataphidini of the subfamily Hormaphidinae are shown. Their gall type, soldier production and gall-cleaning behavior are mapped on the phylogeny. +, − and ± indicate presence of the trait, absence of the trait and some species with the trait while other species without the trait, respectively. Galls of six species examined in this study, N. monzeni and N. distyliicola from Nipponaphidini, C. nekoashi , C. japonica and T. styraci from Cerataphidini, and H. miyabei from Hormaphidini are indicated in bold. Full size image Accumulation of honeydew in open aphid galls Tuberaphis styraci (Cerataphidini) forms large coral-shaped galls on Styrax obassia trees ( Fig. 2a ). Mature galls often harbor over 10,000 insects, and more than half of them may be second instar soldier nymphs specialized for colony defense and gall cleaning [21] , [22] . On the underside of the galls, there are many openings ( Fig. 2b ), through which the soldier nymphs dispose honeydew droplets and other colony wastes [7] , [23] . Of 10 galls of T. styraci we examined, all contained a large amount of wax-coated honeydew droplets ( Fig. 2c ), to which soldier nymphs actively exhibited cleaning behavior by pushing the droplets with their head ( Fig. 2d ). 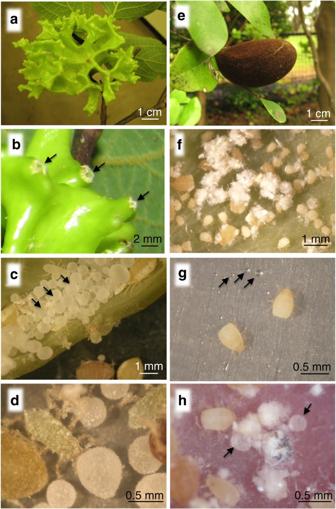Figure 2: Galls ofT. styraciandN. monzeni. (a) A mature gall ofT. styraciformed onS. obassia. (b) Openings located at the projection tips on the underside of a gall ofT. styraci. (c) An inside view of a gall ofT. styraci. Arrows indicate honeydew droplets accumulated in the gall. (d) Gall cleaning behavior of a second-instar soldier nymph ofT. styraci, pushing a honeydew droplet with its head. (e) A mature gall ofN. monzeniformed onD. racemosum. (f) An inside view of an immature gall ofN. monzeni. (g)N. monzeniindividuals placed on an artificial diet. Arrows indicate honeydew droplets excreted by the aphids. (h) An inside view of an immature gall ofN. monzeni. Arrows indicate honeydew droplets. Figure 2: Galls of T. styraci and N. monzeni . ( a ) A mature gall of T. styraci formed on S. obassia . ( b ) Openings located at the projection tips on the underside of a gall of T. styraci . ( c ) An inside view of a gall of T. styraci . Arrows indicate honeydew droplets accumulated in the gall. ( d ) Gall cleaning behavior of a second-instar soldier nymph of T. styraci , pushing a honeydew droplet with its head. ( e ) A mature gall of N. monzeni formed on D. racemosum . ( f ) An inside view of an immature gall of N. monzeni . ( g ) N. monzeni individuals placed on an artificial diet. Arrows indicate honeydew droplets excreted by the aphids. ( h ) An inside view of an immature gall of N. monzeni . Arrows indicate honeydew droplets. Full size image Hamamelistes miyabei (Hormaphidini) forms spiny galls on Hamamelis japonica trees ( Fig. 3a ). Mature galls often contain over 300 insects, wherein monomorphic first-instar nymphs dispose honeydew and other wastes through an opening located at the bottom of the gall [12] . Of eight galls of H. miyabei we inspected, all contained a large mass of wax-coated honeydew ( Fig. 3b ). 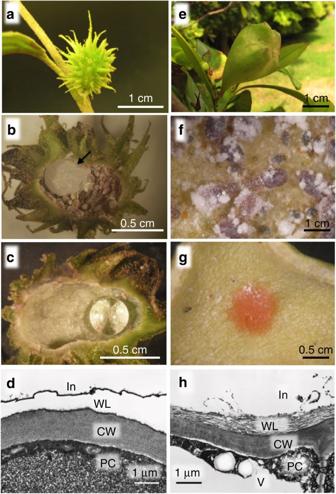Figure 3: Galls ofH. miyabeiandN. distyliicola. (a) A spiny gall ofH. miyabeiformed onH. japonica. (b) An inside view of a gall ofH. miyabeicontaining a number of aphids and a large mass of honeydew (arrow). (c) Hydrophobic inner gall wall ofH. miyabeion which added water forms sphere. (d) Transmission electron microscopy of the inner gall wall ofH. miyabei, in which a well-defined surface wax layer is seen. (e) A fig-shaped gall ofN. distyliicolaformed onD. racemosum. (f) An inside view of a gall ofN. distyliicolacontaining a number of aphids but no honeydew globules. (g) Hydrophilic inner gall wall ofN. distyliicolaon which added water spreads and wets the surface. (h) Transmission electron microscopy of the inner gall wall ofN. distyliicola, where a spongy wax layer is seen. CW, cell wall; In, inner side of the gall; PC, plant cell; V, vacuole; WL, waxy surface layer. Figure 3: Galls of H. miyabei and N. distyliicola . ( a ) A spiny gall of H. miyabei formed on H. japonica . ( b ) An inside view of a gall of H. miyabei containing a number of aphids and a large mass of honeydew (arrow). ( c ) Hydrophobic inner gall wall of H. miyabei on which added water forms sphere. ( d ) Transmission electron microscopy of the inner gall wall of H. miyabei , in which a well-defined surface wax layer is seen. ( e ) A fig-shaped gall of N. distyliicola formed on D. racemosum . ( f ) An inside view of a gall of N. distyliicola containing a number of aphids but no honeydew globules. ( g ) Hydrophilic inner gall wall of N. distyliicola on which added water spreads and wets the surface. ( h ) Transmission electron microscopy of the inner gall wall of N. distyliicola , where a spongy wax layer is seen. CW, cell wall; In, inner side of the gall; PC, plant cell; V, vacuole; WL, waxy surface layer. Full size image These observations indicate that a large number of aphids in the open galls are continuously producing a large amount of honeydew, which must be properly handled and disposed by soldier nymphs for survival and functioning of the aphid colonies [10] . No accumulation of honeydew in closed aphid galls Nipponaphis monzeni (Nipponaphidini) forms closed ball-shaped galls on Distylium racemosum trees ( Fig. 2e ), wherein monomorphic first-instar nymphs attack gall-boring enemies and perform self-sacrificing gall repair [17] , [18] , but exhibit no gall cleaning behavior. The galls rapidly grow during spring–summer, and the mature galls in autumn often contain over 2,000 insects [19] . However, surprisingly, no accumulation of honeydew was observed in both young and mature galls of N. monzeni . Only numerous live insects and powdery aggregates, which consisted mainly of excreted wax and also of shed skins and dry corpses, were found in the closed galls ( Fig. 2f ). The possibility that N. monzeni excretes little honeydew in the galls was rejected by the following observations. When the aphids were placed on an artificial feeding system consisting of a liquid artificial diet sandwiched by Parafilm membranes [24] , a number of honeydew droplets soon appeared around the insects ( Fig. 2g ). Close inspection of young immature galls occasionally identified a small number of honeydew droplets ( Fig. 2h ). Nipponaphis distyliicola (Nipponaphidini) forms closed fig-shaped galls on D. racemosum trees ( Fig. 3e ). Mature galls of N. distyliicola often contain over 700 insects [16] , wherein monomorphic first-instar nymphs attack gall-boring enemies [13] , and as in N. monzeni , no accumulation of honeydew was observed. Only aphids and powdery aggregates were present in the closed galls ( Fig. 3f ). These observations suggest that, in the closed galls of the Nipponaphidini aphids, the insects do excrete a considerable amount of honeydew, but the waste is somehow removed from the closed inner space. Water absorption by closed aphid galls Then, we performed the following field experiments. A small hole was bored on three immature galls of N. monzeni on D. racemosum trees, 1 ml of food dye solution was injected into the galls, and the hole was immediately filled with an adhesive. When we inspected the galls 5 days later, no water remained inside, and the inner bottom wall of the galls was stained in red. Subsequent experiments with more galls revealed that the injected water disappeared within 20 h. To visualize the water absorption routes in detail, we injected 0.5 ml of 0.2% safranin solution into a gall as described above [25] . After 20 h, no solution remained inside the gall, and, strikingly, vein-like staining patterns were clearly observed in the gall wall ( Fig. 4a ). Tissue sectioning of the gall wall unequivocally showed that vascular bundles were selectively stained with safranin ( Fig. 4b ). 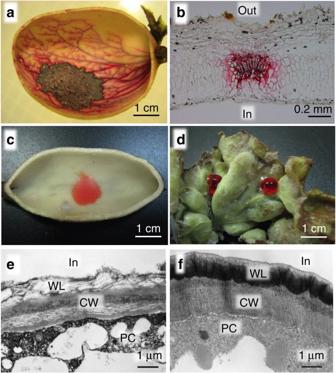Figure 4: Water absorption and histology of galls ofN. monzeniandT. styraci. (a,b) Tracking the route of water absorption in a gall ofN. monzeniby safranin staining. (a) An inside view of the gall 20 h after injection of safranin solution inside. Safranin is precipitated at the bottom of the gall due to water absorption. (b) A histological section of the safranin-injected gall. (c,d) Hydrophobicity of the gall inner surface shown by an addition of food dye water. (c) A gall ofN. monzeni. (d) A gall ofT. styraci. (e,f) Transmission electron microscopy of the inner wall of the galls. (e) A gall ofN. monzeniwith a spongy surface layer. (f) A gall ofT. styraciwith a solid surface layer. CW, cell wall; In, inner side of the gall; Out, outer side of the gall; PC, plant cell; WL, waxy surface layer. Figure 4: Water absorption and histology of galls of N. monzeni and T. styraci . ( a , b ) Tracking the route of water absorption in a gall of N. monzeni by safranin staining. ( a ) An inside view of the gall 20 h after injection of safranin solution inside. Safranin is precipitated at the bottom of the gall due to water absorption. ( b ) A histological section of the safranin-injected gall. ( c , d ) Hydrophobicity of the gall inner surface shown by an addition of food dye water. ( c ) A gall of N. monzeni . ( d ) A gall of T. styraci . ( e , f ) Transmission electron microscopy of the inner wall of the galls. ( e ) A gall of N. monzeni with a spongy surface layer. ( f ) A gall of T. styraci with a solid surface layer. CW, cell wall; In, inner side of the gall; Out, outer side of the gall; PC, plant cell; WL, waxy surface layer. Full size image These results indicate that the gall wall of N. monzeni is capable of absorbing water from inside through the vascular system, and suggest that the honeydew excreted by gall inhabitants is removed by the mechanism. Water absorption driven by water potential of gall wall of N. monzeni What mechanisms are involved in the water absorption by the gall wall of N. monzeni ? A possible mechanism is passive water absorption driven by water potential of the plant tissue, whereas an alternative mechanism is more specific water absorption mediated by water channels such as aquaporins [26] . When water absorption was measured for gall wall preparations in the laboratory, addition of mercury chloride, an aquaporin inhibitor, did not affect the levels of water absorption ( Fig. 5 ). Moreover, a non-water substance, safranin, was efficiently incorporated into the gall tissue ( Fig. 4a ). These observations suggest that aquaporin-mediated water transport is unlikely to be the major mechanism for water absorption by the gall wall of N. monzeni . 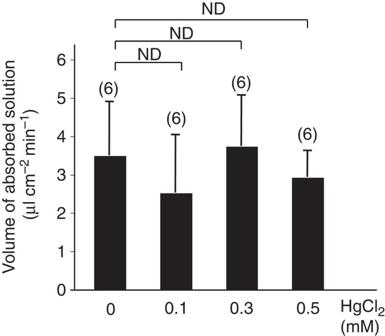Figure 5: Effects of an aquaporin inhibitor on the water absorption by the inner gall wall ofN. monzeni. Means and s.d. are shown with sample sizes in parentheses. ND means no significant difference (generalized linear model;P>0.05). Figure 5: Effects of an aquaporin inhibitor on the water absorption by the inner gall wall of N. monzeni . Means and s.d. are shown with sample sizes in parentheses. ND means no significant difference (generalized linear model; P >0.05). Full size image Next, 58 immature galls of N. monzeni and 10 immature galls of N. distyliicola were subjected to the following field and laboratory experiments. In the field, 1 ml each of distilled water, 2% (58.5 mM) sucrose water, 4% (117 mM) sucrose water and 8% (234 mM) sucrose water was injected into each of 16, 10, 10 and 11 galls of N. monzeni , respectively. Also in the field, 1 ml of distilled water was injected into each of 11 galls of N. distyliicola . In addition, 1 ml of distilled water was injected into each of 11 galls of N. monzeni kept on water bottles in the laboratory. Water remaining in each of the galls was inspected after 20 h. In the distilled water treatment, almost complete absorption (>90%) was observed in 15 of 16 galls of N. monzeni examined in the field ( Fig. 6a ), 5 of 11 galls of N. monzeni examined in the laboratory ( Fig. 6e ) and 4 of 10 galls of N. distyliicola in the field ( Fig. 6f ). In the 2% sucrose water treatment, complete absorption occurred in six galls of N. monzeni , whereas the other four galls exhibited 50–90% absorption ( Fig. 6b ). In the 4% sucrose water treatment, almost complete absorption was found in two galls, whereas the other eight galls exhibited 35–90% absorption ( Fig. 6c ). In the 8% sucrose water treatment, all the 11 galls exhibited little water absorption ( Fig. 6d ). 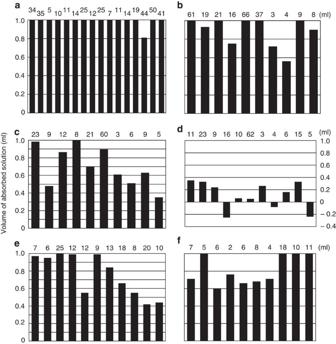Figure 6: Water absorption by galls ofN. monzeniandN. distyliicola. (a) Distilled water in galls ofN. monzeni, field experiment (n=16). (b) Two percentage (58.5 mM) sucrose water in galls ofN. monzeni, field experiment (n=10). (c) Four percentage (117 mM) sucrose water in galls ofN. monzeni, field experiment (n=10). (d) Eight percentage (234 mM) sucrose water in galls ofN. monzeni, field experiment (n=11). (e) Distilled water in galls ofN. monzeni, laboratory experiment (n=11). (f) Distilled water in galls ofN. distyliicola, field experiment (n=10). The number above each column indicates volume (ml) of the gall. Figure 6: Water absorption by galls of N. monzeni and N. distyliicola . ( a ) Distilled water in galls of N. monzeni , field experiment ( n =16). ( b ) Two percentage (58.5 mM) sucrose water in galls of N. monzeni , field experiment ( n =10). ( c ) Four percentage (117 mM) sucrose water in galls of N. monzeni , field experiment ( n =10). ( d ) Eight percentage (234 mM) sucrose water in galls of N. monzeni , field experiment ( n =11). ( e ) Distilled water in galls of N. monzeni , laboratory experiment ( n =11). ( f ) Distilled water in galls of N. distyliicola , field experiment ( n =10). The number above each column indicates volume (ml) of the gall. Full size image These results indicate that the effect of water potential is mainly involved in the water absorption by the gall wall of N. monzeni, and probably in that of N. distyliicola . Water potential quantifies the tendency of water to move from one area to another due to osmosis, gravity, mechanical pressure and matrix effects such as surface tension [26] . Judging from our data, the water potential of the gall wall may be roughly equivalent to the osmotic pressure of 8% (234 mM) sucrose water. Sugar analysis of honeydew samples Of 2 μl of honeydew sample collected from >30 immature galls of N. monzeni , initially 0.5 μl and next 1.0 μl were analysed by liquid chromatography. In both measurements, no distinct peaks were detected for fructose, sucrose, maltose, trehalose and melezitose. The only significant peak was that of glucose. The glucose concentration was estimated as 0.12% (6.7 mM) in the first measurement and as 0.34% (18.9 mM) in the second measurement, respectively ( Supplementary Fig. S2 ). Considering that even 4% (117 mM) sucrose water was efficiently absorbed by the gall wall ( Fig. 6c ), it is expected that honeydew of N. monzeni is readily absorbed by and removed from the aphid gall. No water absorption by open aphid galls As for the open galls of T. styraci , by contrast, no such water absorption was observed. We collected 11 galls of T. styraci , and injected 0.3–1.0 ml of food dye solution depending on the gall size into each of the galls. To minimize the effects of soldiers’ gall cleaning activity, the dye solution was injected into a gall area that had no gall opening. After 20 h, almost the same amount of dye solution was recovered from each of the galls. The gall wall of the area exhibited no dye staining. These results indicate no water absorption by the galls of T. styraci . Hydrophobicity and ultrastructure of gall inner surface Notably, when the dye water was applied to the inner gall surface of N. monzeni , the water immediately spread and wet the surface ( Fig. 4c ). Water droplets placed on the inner gall surface of N. monzeni exhibited a contact angle of 50.7±16.6° (average±s.d., n =12). By contrast, the dye water was repelled by the inner gall surface of T. styraci , forming water spheres ( Fig. 4d ). Water droplets placed on the inner gall surface of T. styraci exhibited a contact angle of 130.8±11.8° ( n =13). Transmission electron microscopy revealed a remarkable structural difference in their gall inner surface: a thick and distinct surface layer, which is presumably made of wax, was observed in the galls of T. styraci ( Fig. 4f ), whereas the layer was thin, reticular and spongy in the galls of N. monzeni ( Fig. 4e ). Interestingly, similar patterns were consistently observed in the galls of other aphid species: hydrophobic inner gall surface exhibiting a water contact angle of 114.0±10.7° ( n =12) with distinct surface layer in the open galls of H. miyabei ( Fig. 3c ) in contrast to hydrophilic inner gall surface exhibiting a water contact angle of 43.4±13.8° ( n =13) with spongy surface layer in the closed galls of N. distyliicola ( Fig. 3g ). Plant-mediated removal of aphid honeydew in closed galls On the basis of these results, we conclude that in N. monzeni (and possibly also in N. distyliicola ), the honeydew excreted by a large number of aphids, which can potentially drown and kill the aphids in the closed space, is absorbed by plant tissue of the gall inner wall, whereby the gall inside is kept dry and safe. Previous studies on a number of Cerataphidini and Hormaphidini aphids consistently reported that soldier nymphs have a pivotal role for removing honeydew and other wastes by their gall cleaning behavior [7] , [9] , [11] , [12] . The plant-mediated honeydew absorption, which entails insect’s manipulation of plant morphogenesis and physiology, is a previously unknown type of gall cleaning. Congenic Cerataphidini aphids forming open and closed galls In general, Cerataphidini aphids form open galls on their specific Styrax trees [5] . For example, Ceratovacuna japonica forms banana-bundle-shaped galls on S. japonicus trees ( Fig. 7a ). Each of 6–12 subgalls has a hollow cavity with a slit opening at the tip ( Fig. 7b ), and contains from 50 to over 100 aphids inside ( Fig. 7c ). In the open galls, C. japonica produces second-instar soldier nymphs, which attack natural enemies as well as perform gall cleaning [27] . Here it is notable that there is an exceptional Cerataphidini species, C. nekoashi , that is congenic with C. japonica but forms closed galls on the same S. japonicus trees ( Fig. 7f ) [15] . Each of 9–13 subgalls comprises a closed cavity without opening and harbors from 50 to over 100 aphids ( Fig. 7g ). The second-instar soldier nymphs of C. nekoashi certainly attack natural enemies, but do not perform gall cleaning [14] . Molecular phylogenetic analysis confirmed that C. japonica and C. nekoashi belong to the same monophyletic group consisting of Pseudoregma / Ceratovacuna species in the Cerataphidini ( Supplementary Fig. S1 ). Hence, comparison between C. japonica and C. nekoashi will provide insights into evolutionary aspects of the open and closed galls. 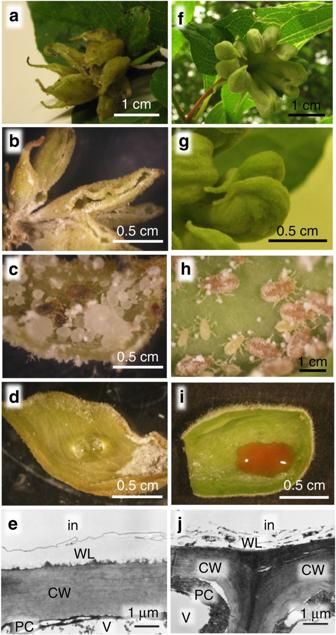Figure 7: Galls ofC. japonicaandC. nekoashi. (a) A banana-shaped gall ofC. japonicawith 12 subgalls formed onStyrax japonicus. (b) Subgalls ofC. japonicawith a slit opening on their tip. (c) An inside view of a subgall ofC. japonicacontaining a number of honeydew droplets and insects. (d) Hydrophobic inner gall wall ofC. japonicaon which added water forms a sphere. (e) Transmission electron microscopy of the inner gall wall ofC. japonica, in which a well-defined surface wax layer is seen. (f) A banana-shaped gall ofC. nekoashiwith 11 subgalls formed onS. japonicus. (g) Closed subgalls ofC. nekoashiwith no opening. (h) An inside view of a subgall ofC. nekoashi, where no honeydew droplets are found despite a number of gall inhabitants. (i) Hydrophilic inner gall wall ofC. nekoashion which added water spreads and wets the surface. (j) Transmission electron microscopy of the inner gall wall ofC. nekoashi, where a spongy surface layer is seen. CW, cell wall; In, inner side of the gall; PC, plant cell; V, vacuole; WL, waxy surface layer. Figure 7: Galls of C. japonica and C. nekoashi . ( a ) A banana-shaped gall of C. japonica with 12 subgalls formed on Styrax japonicus . ( b ) Subgalls of C. japonica with a slit opening on their tip. ( c ) An inside view of a subgall of C. japonica containing a number of honeydew droplets and insects. ( d ) Hydrophobic inner gall wall of C. japonica on which added water forms a sphere. ( e ) Transmission electron microscopy of the inner gall wall of C. japonica , in which a well-defined surface wax layer is seen. ( f ) A banana-shaped gall of C. nekoashi with 11 subgalls formed on S. japonicus . ( g ) Closed subgalls of C. nekoashi with no opening. ( h ) An inside view of a subgall of C. nekoashi , where no honeydew droplets are found despite a number of gall inhabitants. ( i ) Hydrophilic inner gall wall of C. nekoashi on which added water spreads and wets the surface. ( j ) Transmission electron microscopy of the inner gall wall of C. nekoashi , where a spongy surface layer is seen. CW, cell wall; In, inner side of the gall; PC, plant cell; V, vacuole; WL, waxy surface layer. Full size image Water absorption by gall tissue in closed gall of C. nekoashi In total, we found 69 wax-coated honeydew droplets including 61 small ones (<1 mm in diameter) and 8 large ones (1–3 mm in diameter) in 12 open subgalls of C. japonica , and second-instar soldier nymphs were actively pushing and discarding them out through the slit opening ( Fig. 7c ). The inner gall wall was hydrophobic, repelling added water to form spheres with a contact angle of 112.7±7.9° ( n =12) ( Fig. 7d ). Transmission electron microscopy revealed a thick and well-defined surface layer of the inner gall wall, which is presumably made of wax ( Fig. 7e ). By contrast, only five small honeydew droplets (<1 mm in diameter) were detected in 24 closed subgalls of C. nekoashi , although the number of inhabiting aphids was almost the same as in the subgalls of C. japonica ( Fig. 7h ). The inner gall wall was hydrophilic: added water immediately spread and wet the surface, showing a contact angle of 66.5±17.8° ( n =13) ( Fig. 7i ). Transmission electron microscopy revealed a reticular and spongy surface layer of the inner gall wall ( Fig. 7j ). When 0.05 ml of distilled water was injected into each of 16 subgalls from seven galls of C. nekoashi , inspection after 20 h detected no water in the subgalls. These results indicate that, in the aphid tribe Cerataphidini, not only formation of closed galls but also water absorption by gall tissue has evolved in the lineage of C. nekoashi . In this study, we demonstrated that some social aphids form completely closed galls and live socially therein for a considerable period in isolation, these aphids excrete honeydew in their closed galls but little honeydew accumulates in the closed gall cavity, aqueous solution injected into the gall cavity is promptly absorbed by the gall inner wall and removed via the plant vascular system, the water absorption is driven by water potential of the gall tissue, the water-absorbing galls are characterized by not waxy but spongy inner surface layer, the water-absorbing galls have evolved at least twice among the social aphids, and the evolution of water-absorbing galls seems coincident with the evolution of closed galls. Our finding unveils a previously unknown mechanism of gall cleaning, which can be regarded as an ‘extended phenotype’ and a ‘plant-mediated social behavior’ of the social aphids. Here we point out that, among the gall-forming aphids of the subfamily Hormaphidinae, whether they form open galls or closed galls is correlated with an array of seemingly adaptive traits that ecologically function in the social aphid colonies. Namely, some social aphids form open galls, the inner surface of their gall develops a hydrophobic layer that repels water to form honeydew droplets, their soldier nymphs exhibit not only defensive behavior but also cleaning behavior, and the aphid honeydew excreted in the galls is removed by social behavior of the soldier nymphs. By contrast, other social aphids form closed galls, the inner surface of their galls is hydrophilic and absorbs water efficiently, their soldier nymphs may attack enemies but do not clean their galls, and the aphid honeydew excreted in the gall is removed by the plant tissue. The evolutionary link between the closed gall structure and the water-absorbing property seems to make sense biologically, reconciling the otherwise contradictory ecological necessities for the aphid colonies: firm defense against natural enemies versus waste disposal for colony hygiene. In other words, the trade-off between defense and hygiene may have constrained the evolutionary ecology of the galling social aphids. Furthermore, risk of desiccation may also be relevant to the structure of the gall inner surface that is involved in water absorption: the waxy surface layer of open galls may confer resistance to desiccation, whereas the spongy surface layer of closed galls enables water absorption but may lead to vulnerability to desiccation. In N. monzeni , it was reported that, when a hole was bored on the gall wall and gall repairing by soldier nymphs was disrupted, all the artificial open galls died in a few weeks [18] . Not only insects but also terrestrial plants usually develop a waxy layer on their surface, whose principal functions are antidesiccation and defense against pathogens and predators [28] . Many aphids produce a plenty of wax from dorsal wax plates, which prevents contamination with their own honeydew, protects against parasites and predators, provides waterproofing and so on [29] , [30] . The gall-forming Hormaphidinae aphids are notable in that they have evolved several wax-mediated ways to deal with their sticky and putrefactive honeydew waste. In species that form open galls, aphids excrete a plenty of wax and coat their honeydew into marbles, which are easily carried and disposed by soldier nymphs [30] . Moreover, these aphids induce galls with a hydrophobic waxy layer on the inner surface, which facilitates honeydew disposal by soldier nymphs. Notably, the configuration of the wax layer seems different between either aphid lineages or host plant species, on the ground that galls of T. styraci exhibit a wax layer of high electron density whereas galls of C. japonica and H. miyabei are characterized by a wax layer of low electron density ( Figs 3d , 4f and 7e ). In species that form closed galls, by contrast, aphids induce galls with a hydrophilic spongy layer on the inner surface, which enables honeydew removal by absorption via plant vascular system. In addition, our honeydew composition analyses ( Supplementary Fig. S2 ) revealed the following patterns. Firstly, sugar quantities in the honeydew samples were in the order of a free-living aphid ( Aphis craccivora ) >a gall-forming non-social aphid ( Prociphilus ligustrifoliae ) >a gall-forming social aphid ( T. styraci ) >a social aphid that forms water-absorbing closed galls ( N. monzeni ). Second, although plant phloem sap is generally sucrose-rich [20] , the sugar compositions in the honeydew samples were unexpectedly devoid of sucrose, which was particularly conspicuous in gall-forming social aphids including N. monzeni . Lastly, these gall-forming social aphids generally excrete a plenty of wax in their galls, and thus the low sugar concentrations in the honeydew of gall-forming social aphids may be attributable to consumption of sucrose for wax production. On the basis of these results and rationales, although speculative, we propose a hypothesis that the wax production by gall-forming social aphids may contribute to their waste disposal in different ways: in species forming open galls, for making wax-coated honeydew droplets to facilitate soldier-mediated waste disposal; and in species forming closed galls, for excretion of low-osmotic honeydew to facilitate plant-mediated waste removal. An alternative hypothesis is that the social aphids forming closed galls may excrete low-osmotic honeydew wherein sugars are polymerized into polysaccharides. In general, social insect colonies cannot persist for a considerable period in isolation except for the inactive hibernation period, because they constantly require a large amount of food from the environment and also produce a large amount of wastes to be disposed outside. In the galling social aphids, by contrast, their plant-made nests directly provide the plant sap diet, the major component of their wastes is aqueous solution, and these peculiar ecological traits must have enabled some of them to evolve a unique strategy of social living in completely closed galls. Materials Galls of N. monzeni formed on D. racemosum trees were experimentally manipulated and studied at Shinkiba, Tokyo, Japan, from April to June in 2007 to 2012. After a series of experiments, the galls were collected, brought to the laboratory at Tsukuba, Ibaraki, Japan, and subjected to further analyses. Galls of other social aphids examined in this study are listed in Supplementary Table S1 . DNA sequencing and molecular phylogenetic analysis PCR, cloning and sequencing of a 1.6 kb mitochondrial DNA segment containing small subunit rRNA, tRNA-Val and large subunit rRNA genes were performed as described [31] . Accession numbers of the DNA sequences either determined in this study or used for the following phylogenetic analysis are listed in Supplementary Table S2 . A multiple alignment of the nucleotide sequences was generated using the program Clustal W [32] . Aligned nucleotide sites containing gaps were removed from the data set, and the final alignment was inspected and corrected manually. Phylogenetic analyses were conducted by maximum likelihood (ML), maximum parsimony and Bayesian (BA) methods using the programs RAxML 7.0.0 [33] , PAUP 4.0b10 [34] and MrBayes 3.1.2 [35] , respectively. Bootstrap tests were performed with 1,000 samplings for the ML and maximum parsimony. Posterior probabilities were estimated for BA. For the ML and BA analyses, the substitution model was chosen on the basis of the Akaike information criterion with the program jModeltest 0.1.1 [36] , which selected the GTR+I+G model. Experimental manipulation of galls A small 2 × 2 mm square hole was bored on the wall of N. monzeni galls in the field using a fine edge of a chisel. From the hole, 1 ml of food dye water (0.2% Food Red No. 102, Kyoritsu Foods), distilled water or sucrose water was injected into the gall cavity using a 5-ml syringe with a 22G needle (Terumo Co.). Then the hole was immediately filled with an adhesive (Wood Glue, Konishi Co., Ltd; consisting mainly of 41% polyvinyl acetate). For the laboratory experiments, galls of N. monzeni formed on twigs of D. racemosum were brought to the laboratory, and the twigs were put in water bottles during the experiments. Similarly, galls of T. styraci formed on twigs of S. obassia were collected in the field, and the twigs were kept in water bottles during the laboratory experiments. In the water absorption experiments, 1 ml of food dye water was injected from an opening into the gall cavity. After 20 h, the injected solutions were recovered and quantified. In the staining experiment, 0.5 ml of 0.2% safranin solution was injected into a N. monzeni gall as described above. The gall was inspected after 20 h, and frozen sections (16 μm thick) of the gall tissue were made on a cryostat (HM-505E, Carl Zeiss), mounted on glass slides and observed under a light microscope. Aquaporin inhibition assay Six galls of N. monzeni were collected on 5 June 2008, brought to the laboratory and subjected to the experiment. Four 1 × 1 cm pieces of the gall wall were cut out of each gall and placed in a plastic chamber. Onto inner side of the gall pieces, 0.1 ml of distilled water containing either 0 mM, 0.1, 0.3 or 0.5 mM mercury chloride was placed and kept at room temperature. Simultaneously, 0.1 ml of distilled water containing either 0, 0.1, 0.3 or 0.5 mM mercury chloride was placed on a strip of Parafilm membrane in the same chamber to correct the evaporation loss of water. Zhang and Tyerman [37] reported that 0.1 mM mercury chloride was sufficient to inhibit the water channel activity of aquaporins in plant tissues. Three minutes later, the solutions were recovered from the gall pieces and the Parafilm membrane, and weighed on a microbalance. The amount of absorbed water was calculated by (water loss on the gall tissue)−(water loss on the parafilm membrane) in terms of milliliter given a specific gravity of 1. The data were statistically analysed by the software R v. 2.7.2 [38] . Honeydew analysis Wax-coated honeydew droplets were occasionally found in small immature galls of N. monzeni . From >30 immature galls, 2 μl of honeydew was collected using a fine brush and stored in a plastic tube at −80 °C until analysis. Honeydew samples from the other aphid species are listed in Supplementary Table S3 . The honeydew samples were analysed by high-performance liquid chromatography essentially as described [39] . A mixture of six sugar standards (glucose and fructose as monosaccharide, sucrose, maltose and trehalose as disaccharide, and melezitose as trisaccharide) was used for identification and quantification of sugars in the honeydew samples. Electron microscopy Plant tissue specimens of aphid galls were prefixed by 2.5% glutaraldehyde in 0.1 M sodium phosphate buffer (pH 7.2) at 4 °C overnight, and postfixed by 2% osmium tetroxide at 4 °C for 120 min. After dehydration through an ethanol series, the materials were embedded in Spurr resin and cut into ultrathin sections (70 nm thick). The sections were stained with uranyl acetate and lead citrate, and observed with a transmission electron microscope (H-7000; Hitachi). Contact angle measurement Ten microlitre of distilled water was placed on the center of a small piece of inner gall surface, and a digital photograph was taken from a horizontal direction as described [30] . A contact angle between the water droplet and the gall wall was measured manually by using a protractor. In general, the surface is regarded as hydrophobic if the contact angle is >90°, and as hydrophilic if it is <90°. How to cite this article: Kutsukake, M. et al. An insect-induced novel plant phenotype for sustaining social life in a closed system. Nat. Commun. 3:1187 doi: 10.1038/ncomms2187 (2012).